Distinct modes of DNA accessibility in plant chromatin The accessibility of DNA to regulatory proteins is a major property of the chromatin environment that favours or hinders transcription. Recent studies in flies reported that H3K9me2-marked heterochromatin is accessible while H3K27me3-marked chromatin forms extensive domains of low accessibility. Here we show that plants regulate DNA accessibility differently. H3K9me2-marked heterochromatin is the least accessible in the Arabidopsis thaliana genome, and H3K27me3-marked chromatin also has low accessibility. We see that very long genes without H3K9me2 or H3K27me3 are often inaccessible and generated significantly lower amounts of antisense transcripts than other genes, suggesting that reduced accessibility is associated with reduced recognition of alternative promoters. Low accessibility of H3K9me2-marked heterochromatin and long genes depend on cytosine methylation, explaining why chromatin accessibility differs between plants and flies. Together, we conclude that restriction of DNA accessibility is a local property of chromatin and not necessarily a consequence of microscopically visible compaction. In eukaryotes, DNA is wrapped around histone octamers forming the basic ‘beads-on-a-string’ structure of nucleosome arrays of chromatin. This 10 nm nucleosomal fiber can assemble into various higher-order structures. Chromatin organization differs greatly between genome regions, and mechanisms that cause local differences in chromatin include, among others, histone modifications, the insertion of histone variants, and nucleosome mobilization by chromatin-remodelling complexes [1] , [2] , [3] . A well-characterized type of chromatin is pericentromeric heterochromatin, which is typically enriched for repetitive sequences and transposable elements (TEs) and remains cytologically condensed even during interphase [4] . Histones in pericentromeric heterochromatin are hypoacetylated and enriched for methylation at lysine 9 of histone H3 (H3K9me2/3). Another well-characterized chromatin state is established by polycomb group (PcG) proteins, which are major regulators of developmentally controlled gene expression in animals and plants [5] , [6] . Polycomb repressive complex 2 (PRC2) tri-methylates H3K27, which in turn assists other PcG protein complexes such as PRC1 to introduce additional histone modifications. H3K27me3 often forms extensive domains in animals, but H3K27me3 regions are largely restricted to single-gene bodies in Arabidopsis [7] , [8] , [9] . Cytological identification of stably condensed chromatin has led to the assumption that condensed chromatin is static and prevents exchange of chromatin components and access of proteins to DNA. The view of higher-order structure as a regulator of accessibility, however, has been challenged by measurements of diffusional motilities of nuclear proteins. Proteins can readily diffuse even into highly condensed heterochromatin [10] , [11] , [12] , and inert diffusion probes of the size of large protein complexes readily entered condensed chromatin [13] , [14] . Similarly, a recent study of genome-wide DNA accessibility in Drosophila using M.Sss I methylation footprinting questions the view of greatly reduced accessibility of heterochromatin: DNA in chromatin carrying H3K9me2 seems to be as accessible as the rest of the genome [15] . Thus, higher-order folding and microscopically visible compaction of chromatin per se do not prevent access by nuclear proteins. It is possible that accessibility is mainly controlled locally by interactions of neighboring nucleosomes [16] . It is of great importance to discover determinants of DNA accessibility to nuclear proteins and the relation to cytological chromatin compaction. In the model plant A. thaliana , cytologically condensed heterochromatin is considered to be of low complexity mostly comprising centromeric and pericentromeric sequences enriched in H3K9me2 and 5-cytosine DNA methylation [17] . We exploited this particular chromatin architecture to profile genome-wide DNA accessibility using DNase I sensitivity assays coupled to genome tiling microarrays. In contrast to the situation in Drosophila , the least accessible regions in the Arabidopsis genome were pericentromeric heterochromatin marked by H3K9me2 and DNA methylation. Euchromatic and gene-dense chromosome arms were generally accessible but interrupted by isolated, inaccessible chromatin islands that lacked H3K9me2. Instead, these regions often comprised PcG protein targets or very long genes with high genic DNA methylation. Although DNA accessibility was generally negatively correlated with transcription, the group of very long and DNase I inaccessible genes were inaccessible despite being transcribed. As reduced accessibility of pericentromeric heterochromatin and long inaccessible genes required DNA methylation, it appears that PcG proteins and DNA methylation establish inaccessible chromatin in plants. Pericentromeric chromatin forms inaccessible regions Differential accessibility of different chromosomal regions is not well understood. To better understand genomic DNA accessibility, we profiled global DNA inaccessibility in A. thaliana using chromatin DNase I hypo-sensitivity as a functional read-out. The rationale for our approach was that limited digestion with DNase I will generate small DNA fragments from accessible chromosome regions and larger fragments from less accessible regions, allowing separation by size-fractionation methods. Large DNA fragments were labelled and hybridized to genomic DNA tiling arrays ( Fig. 1 ; see Methods section for details). To validate outcomes of this method, we compared microarray-derived inaccessibility scores to results of independent DNase I-PCR experiments without size fractionation for genomic fragments at two pericentromeric TE genes, two active genes and twelve fragments at genes of high inaccessibility ( Supplementary Fig. S1 ). DNase I-PCR and DNase I-chip-derived DNA inaccessibility values agreed well, demonstrating the applicability of the array-based profiling method. 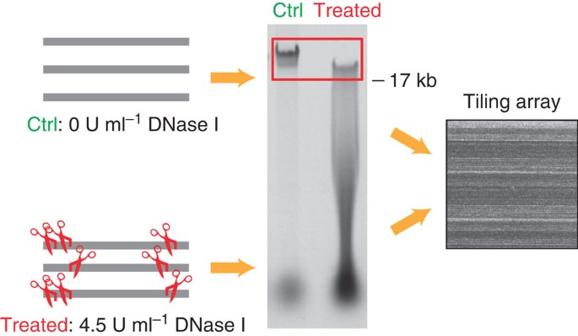Figure 1: Profiling DNA accessibility by DNase I-chip. Chromatin was partially digested with DNase I. Digested (red) and control (green) DNA fragments were hybridized onto microarrays. Figure 1: Profiling DNA accessibility by DNase I-chip. Chromatin was partially digested with DNase I. Digested (red) and control (green) DNA fragments were hybridized onto microarrays. Full size image DNA accessibility over the genome exhibited a wide dynamic range between the least and most accessible sites, and forms a continuous distribution with a pronounced tail toward high inaccessibility ( Fig. 2a ). We define the chromatin regions that are least sensitive to DNase I as ‘inaccessible regions’. We identified 388 extended inaccessible regions of a total length of over 22 Mb. Conversely, we also identified 1957 hyper-accessible regions of a total length of 350 kb (see Methods). The hyper-accessible and inaccessible regions contained contrasting sets of genomic features (protein-coding genes, pseudogenes, TE genes, TEs; classification according to the Arabidopsis genome annotation) ( Fig. 2b ). The inaccessible regions comprised ~17,600 annotated genomic features, of which about 90% were TE genes, TEs and pseudogenes, and only a minor fraction (<10%) were protein-coding genes. In contrast, the hyper-accessible regions comprised almost exclusively protein-coding genes (98%) ( Fig. 2b ). Consistently, the density of inaccessible regions across the genome correlated positively with the TE density (Spearman’s correlation per chromosome=0.90±0.0, P -value=1 × 10 −16 ) but negatively with protein-coding gene density (Spearman’s correlation per chromosome=−0.86±0.04, P -value=1 × 10 −16 ) ( Fig. 2c ; Supplementary Fig. S2 ). Conversely, a majority (~93%) of permanently silenced TE genes reside in highly inaccessible chromatin. Notably, the 22 Mb inaccessible regions comprised about 16% of the Arabidopsis genome (~135 Mb [18] ), which closely matches results from previous cytological studies that estimated a chromocenter-localized heterochromatin fraction of 15–17% in Arabidopsis [19] , [20] . These results identify pericentromeric heterochromatin as a major component of inaccessible chromatin in Arabidopsis . 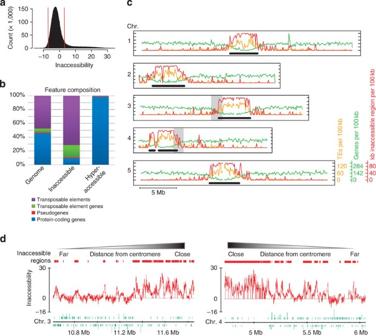Figure 2: Pericentromeric heterochromatin is least accessible. (a) Distribution of DNA inaccessibility scores. Vertical lines represent thresholds for the selection of hyper- and hypo-accessible regions. (b) Distribution of genomic features in inaccessible and hyper-accessible regions. (c) Density of inaccessible regions (red), protein-coding genes (green) and TEs (yellow) along chromosomes. Bars mark centromeric and pericentromeric heterochromatin. (d) Details of inaccessibility profiles at borders of pericentromeric heterochromatin (shaded blocks inc). Green bars represent annotated genes. Figure 2: Pericentromeric heterochromatin is least accessible. ( a ) Distribution of DNA inaccessibility scores. Vertical lines represent thresholds for the selection of hyper- and hypo-accessible regions. ( b ) Distribution of genomic features in inaccessible and hyper-accessible regions. ( c ) Density of inaccessible regions (red), protein-coding genes (green) and TEs (yellow) along chromosomes. Bars mark centromeric and pericentromeric heterochromatin. ( d ) Details of inaccessibility profiles at borders of pericentromeric heterochromatin (shaded blocks in c ). Green bars represent annotated genes. Full size image The hetero-to-euchromatin transition is gradual Traditionally, Arabidopsis heterochromatin regions were probed by fluorescence in situ hybridization experiments [21] , [22] , which have limited resolution and throughput. Here, we attempted to define the borders of pericentromeric heterochromatin by an original definition—condensed chromatin regions with limited accessibility [23] —using the DNA inaccessibility measures as a functional proxy. Interestingly, however, pericentromeric sequences ( Fig. 2c , black bars) were highly enriched for inaccessible chromatin regions but did not form uniform inaccessible blocks. Rather than forming sharp, step-like borders, the transition between inaccessible pericentromeric heterochromatin and accessible euchromatin arms was gradual. Inaccessible regions were more often interrupted by accessible regions with increasing distance from centromeres ( Fig. 2d ). These increasing interruptions mirrored the gradual increase in protein-coding gene density and the gradual decrease in TE density ( Fig. 2c ). In other words, inaccessible pericentromeric heterochromatin in Arabidopsis is not demarcated by sharp borders but invades into neighbouring accessible sequences. H3K9me2 is a major modification of inaccessible chromatin Arabidopsis pericentromeric regions are enriched for H3K9me2 and DNA-methylation [24] , [25] . Contrasting to the findings in flies, where H3K9me2-marked heterochromatin is as accessible as the rest of the genome, the pericentromeric enrichment of Arabidopsis inaccessible regions in our data suggests that H3K9me2 is associated with inaccessible chromatin in Arabidopsis . We, therefore, explored the relationship between DNA accessibility and H3K9me2. Globally, DNA inaccessibility correlated strongly and positively with H3K9me2 ( Fig. 3a ; Spearman’s correlation per chromosome=0.60±0.02, P -value=2.2 × 10 −16 ). Nevertheless, some sequences were highly accessible despite high H3K9me2 coverage (cloud below the diagonal in Fig. 3a ). Manual inspection of several of these regions revealed that they usually contain small TE genes that are embedded in accessible chromatin environments of active genes. Next, we explored the H3K9me2 distribution in proximities of all genes dependent on their different inaccessibility levels, quantified as a gene-wise inaccessibility score (see Methods). Of note, genes with high inaccessibility scores can reside outside of inaccessible regions, which were defined as inaccessible chromatin domains of extended lengths, not including short stretches of inaccessible chromatin. We grouped all genes by increasing inaccessibility, and plotted for each bin an averaged H3K9me2 profile in the gene proximities ( Fig. 3b ). Clearly, the least accessible genes showed substantial H3K9me2 enrichment ( Fig. 3b , bin 10, pink) both at gene bodies and at the proximal flanking sequences. In contrast, more accessible genes lacked H3K9me2. This indicates that H3K9me2 is an important component of the least accessible chromatin in Arabidopsis , much in contrast to the situation in flies. 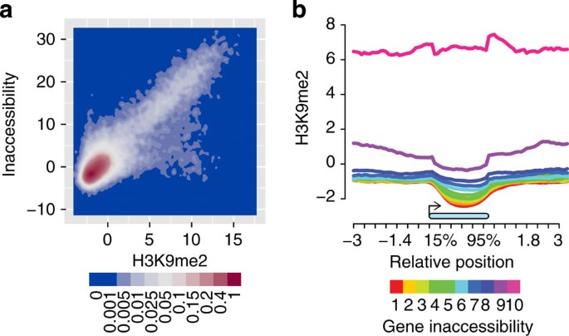Figure 3: Least accessible chromatin is rich in H3K9me2. (a) Distribution of DNA accessibility scores and H3K9me2 enrichments (red, high data point density; blue, low density). (b) H3K9me2 profiles across genes grouped by accessibility. Figure 3: Least accessible chromatin is rich in H3K9me2. ( a ) Distribution of DNA accessibility scores and H3K9me2 enrichments (red, high data point density; blue, low density). ( b ) H3K9me2 profiles across genes grouped by accessibility. Full size image Interestingly, genes in the second least accessible bin generally lacked H3K9me2 ( Fig. 3b , bin 9, purple and Supplementary Fig. S3 ). This indicates that accessibility can be reduced without involving the canonical heterochromatic H3K9me2. In contrast to the pericentromeric localization of most of the H3K9me2-marked inaccessible genes, the inaccessible genes without H3K9me2 were usually located in the inaccessible islands interspersed on the gene-rich chromosome arms ( Fig. 2c ). Together, we identified two major distinct types of inaccessible chromatin. The first type comprises pericentromeric heterochromatin and is associated with high levels of H3K9me2 and DNA methylation; the second type is scattered along the chromosome arms and does not carry H3K9me2. Active genes are most accessible DNA inaccessibility is thought to restrict recognition of DNA templates by regulatory proteins and thus to hinder transcription while accessible chromatin structures may facilitate transcription [15] , [26] . It is also possible that increased DNA accessibility is a consequence of transcriptional activity. In our data set, DNA accessibility and transcript levels had a positive correlation (Spearman’s correlation per chromosome=0.38±0.02, P -value=2.2 × 10 −16 ). The relation between transcript levels and DNA inaccessibility was gradual rather than step-like ( Fig. 4a ), suggesting that increased transcription correlates with a gradual increase in DNA accessibility and not with a switch-like, sharp increase. Next, we tested how far effects of transcription on DNA accessibility extend from the transcription unit. Averaged DNA inaccessibility profiles across genes were plotted after grouping genes into four bins of increasing transcript abundance ( Fig. 4b ). Bodies and flanking sequences of inactive genes showed high inaccessibility signals, suggesting that such genes often reside in neighbourhoods of low DNA accessibility ( Fig. 4b , red, green, bins 1–2). In contrast, active genes had low inaccessibility signals ( Fig. 4b , cyan, purple, bins 3–4). Notably, accessibility was considerably higher at gene bodies than at flanking sequences. This indicates that the increase of DNA accessibility associated with transcription acts locally and does not extend far from the transcription unit. 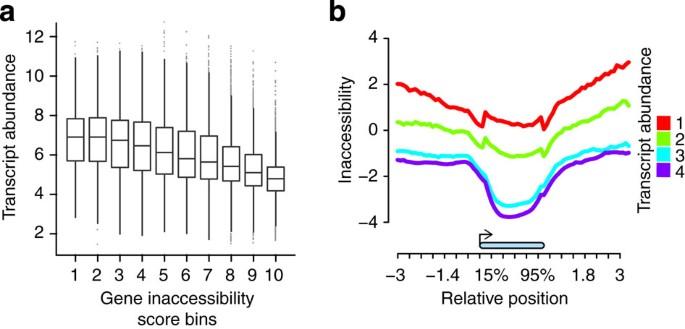Figure 4: Inactive genes are less accessible than active genes. (a) Relation between transcript abundance and DNA accessibility. (b) DNA accessibility profiles across genes grouped by expression. Figure 4: Inactive genes are less accessible than active genes. ( a ) Relation between transcript abundance and DNA accessibility. ( b ) DNA accessibility profiles across genes grouped by expression. Full size image PcG targets have reduced accessibility To identify mechanisms that further reduce accessibility of inactive genes, we next focused on PcG proteins, which form a major class of transcriptional repressors. PcG proteins are essential for normal development but the mechanisms by which they repress target gene transcription are not well understood. About two decades ago, it was proposed that animal PcG proteins repress transcription by chromatin compaction and reducing DNA accessibility, but only recently evidence supporting this view has started to accumulate for animal systems [15] , [27] , [28] , [29] . As patterns of H3K27me3 enrichment and PcG protein complex composition are only partially conserved between plants and animals [5] , it is not clear whether in plants repression by PcG proteins involves chromatin compaction. Here, we asked whether plant PcG target genes contributed to the set of inaccessible genes. Indeed, nearly half (46.2%) of the genes in inaccessible regions without H3K9me2 were PcG targets. Levels of H3K27me3, the hallmark of PcG repression, showed positive correlation at gene level with DNA inaccessibility ( Fig. 5a ; see Fig. 5b for an example). Specifically, H3K27me3 was clearly enriched in bodies of genes with low accessibility. H3K27me3 was only partially enriched in the least accessible genes as this group is dominated by genes marked by H3K9me2, which together with DNA methylation excludes H3K27me3 [7] , [9] , [30] . Notably, PcG targets were significantly less accessible than other inactive genes lacking H3K9me2 ( P -value=2.2 × 10 −16 ) ( Fig. 5c ), indicating that the reduced accessibility of the PcG targets is not a mere consequence of repressed transcription. These results reveal that gene repression by plant PcG proteins is associated with locally reduced DNA accessibility. 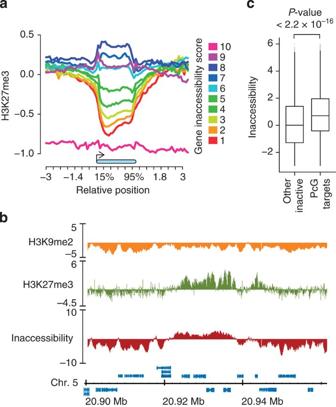Figure 5: Targets of Polycomb group proteins have low accessibility. (a) H3K27me3 profiles across genes grouped by accessibility. (b) Epigenome profiles along a region on chromosome 5 including several PcG target genes. (c) Inaccessibility of other inactive genes and PcG targets (P-value was from Wilcoxon’s-signed rank test, one-tail). Figure 5: Targets of Polycomb group proteins have low accessibility. ( a ) H3K27me3 profiles across genes grouped by accessibility. ( b ) Epigenome profiles along a region on chromosome 5 including several PcG target genes. ( c ) Inaccessibility of other inactive genes and PcG targets ( P -value was from Wilcoxon’s-signed rank test, one-tail). Full size image Long genes methylated in the gene body are inaccessible In addition to the two classes of inaccessible genes defined by H3K9me2 or H3K27me3, we identified a third class, which carries neither H3K9me2 nor H3K27me3 ( Fig. 6a–c ; see Fig. 6d for an example). Genes in this class were often very long ( Fig. 6d ; Supplementary Fig. S4 ); nearly half of the inaccessible genes lacking both H3K9me2 and H3K27me3 belonged to the 5% longest of all genes. We next investigated whether these long genes had low accessibility because of repressed transcription by comparing transcript levels of the different classes of inaccessible genes. Consistent with the global correlation between transcription and accessibility, inaccessible genes with H3K9me2 or H3K27me3, and genes from hyper-accessible regions (hyper-accessible genes) had low and high transcript levels, respectively ( Fig. 6e ). Surprisingly, the long inaccessible genes were not silenced but expressed at levels comparable to the hyper-accessible genes ( Fig. 6e ), suggesting that this type of chromatin compaction is not associated with canonical repression of transcription. In addition, this observation demonstrates that transcription does not inevitably cause increased DNA accessibility. 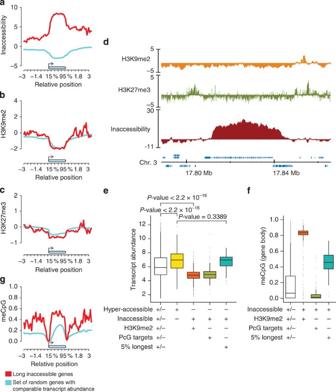Figure 6: The longest genes have low accessibility even when transcribed. (a–c,g) Inaccessibility, H3K9me2, H3K27me3 and methylated CpG (meCpG) profiles across long inaccessible genes (red) and accessible genes with similar sense transcript levels (azure). (d) Epigenome profiles along a region on chromosome 3 including a very-long gene. (e) Transcript abundance of genes grouped by accessibility (P-values from Wilcoxon’s-signed rank test, two-tail). (f) Cytosine methylation in -Cytosine-phosphate-Guanine- (CpG) contexts in gene bodies. Figure 6: The longest genes have low accessibility even when transcribed. ( a – c , g ) Inaccessibility, H3K9me2, H3K27me3 and methylated CpG (meCpG) profiles across long inaccessible genes (red) and accessible genes with similar sense transcript levels (azure). ( d ) Epigenome profiles along a region on chromosome 3 including a very-long gene. ( e ) Transcript abundance of genes grouped by accessibility ( P -values from Wilcoxon’s-signed rank test, two-tail). ( f ) Cytosine methylation in -Cytosine-phosphate-Guanine- (CpG) contexts in gene bodies. Full size image It has been reported that long Arabidopsis genes are enriched for genic DNA methylation especially toward the 3′-end [31] , [32] , [33] . Confirming previous observations, cytosine methylation in CpG contexts in gene bodies of long inaccessible genes was significantly above the genome median ( P -value=2.2 × 10 −16 ) but lower than methylation in inaccessible genes with H3K9me2 ( P -value=2.2 × 10 −16 ; Fig. 6f–g ). Cytosine methylation was not increased in other sequence contexts or in promoters of these long inaccessible genes ( Supplementary Fig. S5 ). DNA methylation in gene bodies but not promoters also coincided with higher DNA inaccessibility in gene bodies than in promoters (compare Fig. 6a ). Thus, it appeared possible that DNA methylation on CpG nucleotides in gene bodies contributes to reduced DNA accessibility. Inaccessibility of TE and long genes requires DNA methylation We have found that H3K9me2-marked pericentromeric heterochromatin is inaccessible in the Arabidopsis genome. This was in contrast to flies, where H3K9me2-marked heterochromatin is not particular inaccessible. We, therefore, considered molecular mechanisms that could contribute to the low accessibility of H3K9me2-marked chromatin in Arabidopsis . As both H3K9me2-marked genes and long inaccessible genes were highly methylated at cytosines [25] , [32] ( Fig. 6g ; Supplementary Fig. S5 ) but DNA methylation is very low in flies [34] , we hypothesized that cytosine methylation contributes to low DNA accessibility in Arabidopsis . This hypothesis was tested by treating seedlings with 5-azacytidine, which is an established method to deplete the Arabidopsis genome of cytosine methylation [35] , [36] , [37] . In treated seedlings, accessibility of tested long genes and TE genes increased strongly and became similar to that of accessible active genes ( Fig. 7a ). Similarly, genetic reduction of cytosine methylation in a ddm1 mutant [38] , [39] , [40] also caused increased accessibility of the tested fragments ( Supplementary Fig. S6 ). Importantly, only one out of the six inaccessible genes tested showed increased transcript abundance upon 5-azacytidine treatment ( Fig. 7b ). Thus, the general increase in accessibility was not a mere consequence of transcription activation. These results indicate that cytosine methylation is required to reduce the accessibility of long genes and TE genes. 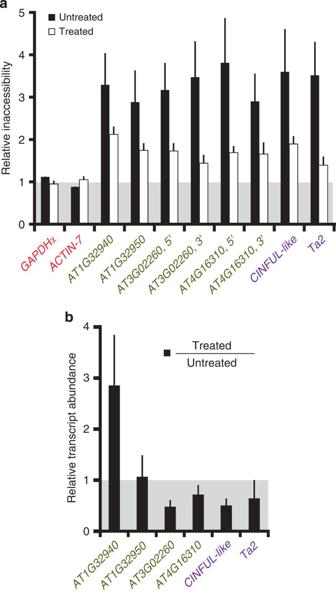Figure 7: Low accessibility of long genes requires DNA methylation. (a) DNA accessibility at accessible active (red), inaccessible long active (green) and inaccessible silent genes (purple) after treatment with 5-azacytidine to reduce DNA methylation. (b) Effect of 5-azacytidine treatment on transcript levels. (a) and (b) show means of three biological replicates. Error bars show s.e.m.. Figure 7: Low accessibility of long genes requires DNA methylation. ( a ) DNA accessibility at accessible active (red), inaccessible long active (green) and inaccessible silent genes (purple) after treatment with 5-azacytidine to reduce DNA methylation. ( b ) Effect of 5-azacytidine treatment on transcript levels. ( a ) and ( b ) show means of three biological replicates. Error bars show s.e.m.. Full size image Inaccessible long genes have reduced antisense transcription It has been proposed that genic DNA methylation could function to repress intragenic cryptic promoters [31] . We, therefore, considered that the reduced DNA accessibility mediated by CpG methylation at the long inaccessible genes is associated with repression of cryptic promoters in the gene body. We reasoned that antisense transcript levels could be used as proxy for the activity of alternative promoters and tested whether the low accessibility of the long genes was associated with low antisense transcript levels. Indeed, antisense transcript levels of long inaccessible genes were significantly below the genome average ( Fig. 8a ; P -value=5.5 × 10 −8 ). This is in stark contrast to the abundance of sense transcripts, which were considerably above genome average ( Fig. 6b ). Inaccessible long genes had significantly lower antisense transcript levels than other long genes ( P -value=3.3 × 10 −6 ) ( Fig. 8b , left). In contrast, inaccessible and accessible long genes had sense transcript levels not significantly different from each other ( P -value=0.053) ( Fig. 8b , right). Therefore, the reduced accessibility seems to be preferentially associated with repression of transcription from alternative promoters. Identical results were also obtained using publically available strand-specific RNA sequencing data [41] ( Supplementary Fig. S7 ). Genome-wide, higher accessibility of genes also seems to allow more antisense transcription. For the hyper-accessible genes, not only levels of sense ( Fig. 6b ) but also antisense transcripts were significantly higher than the genome median ( P -value=5.9 × 10 -5 ; Fig. 8a ). Together, these results suggest that transcription from intragenic promoters is not strongly controlled for most active genes but is reduced at long inaccessible genes. 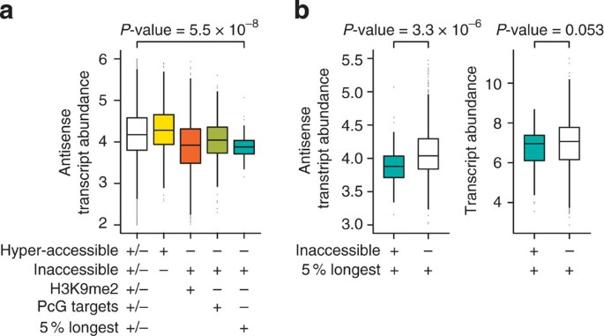Figure 8: Inaccessible long genes generate low levels of antisense transcripts. (a) Levels of antisense transcripts in genes grouped by accessibility. (b) Antisense and sense transcript levels in inaccessible and accessible long genes.P-values were from Wilcoxon’s-signed rank test, one-tail. Figure 8: Inaccessible long genes generate low levels of antisense transcripts. ( a ) Levels of antisense transcripts in genes grouped by accessibility. ( b ) Antisense and sense transcript levels in inaccessible and accessible long genes. P -values were from Wilcoxon’s-signed rank test, one-tail. Full size image DNA accessibility is thought to be important for the regulation of transcriptional control, and it has been proposed that a major function of the multiple combinations of histone modifications is to fine-tune accessibility of the DNA [42] . As constitutive heterochromatin contains mostly silent sequences that remain densely compacted even during interphase [4] , it was generally thought to strongly restrict the access of proteins to DNA. However, several studies have now suggested that this view might be an oversimplification. Not only do various high-molecular weight probes and proteins readily enter heterochromatin [10] , [11] , [12] , [13] , [14] , but also transcription of repetitive sequences by specific RNA polymerases is required for methylation of H3K9 and heterochromatin assembly [43] . It is possible that bursts of transcription occur particularly during S-phase offering an explanation to reconcile the conflicting concepts of transcriptional repression and active transcription in heterochromatin [44] , [45] , [46] . More recently, the prevailing concept of constitutive heterochromatin being inaccessible was again challenged by the finding that heterochromatin in Drosophila was not less accessible than the genome average [15] . In stark contrast, our data revealed that H3K9me2-marked heterochromatin regions in Arabidopsis have by far the lowest DNase I sensitivity in the genome. In contrast to flies, where H3K9me2 and H3K9me3 are both enriched in constitutive heterochromatin; in Arabidopsis only H3K9me2 is heterochromatic while H3K9me3 is present in the euchromatin. Future work must address how H3K9me3 differentially affects fly heterochromatin and Arabidopsis euchromatin. In Arabidopsis but not in flies, H3K9me2-marked heterochromatin is also rich in 5-cytosine DNA methylation [25] . While we found that DNA methylation is required for low accessibility of several tested loci, DNA methylation was reported to be only partially required for formation of heterochromatic chromocenters [19] . These findings support the notion that microscopically visible compaction such as in heterochromatic chromocenters per se does not greatly restrict accessibility but that DNA accessibility is instead mostly defined at a lower organisational level of chromatin [16] . Therefore, compaction at a cytological scale as visible by microscopy should be differentiated from reduced accessibility, which is established locally and might act mostly at the scale of neighbouring nucleosomes. Similar to repression of sequences in constitutive heterochromatin, silencing of genes targeted by PcG proteins was proposed to result in reduced accessibility. Indeed, long-distance chromatin contacts establish microscopically visible compaction of PcG target genes in Drosophila [47] , and in vitro experiments had suggested that fly PRC1 can compact nucleosome arrays [48] . More recently, it was reported that PcG protein targeting reduces DNA accessibility in Drosophila [15] . In plants, the PcG protein system is partially conserved, but important differences to animals exist [5] . In particular, a strict homolog of PRC1 seems absent and PcG targeting does not usually manifest itself in patterns similar to the whole chromosome repression of Xi or long-range repression of coregulated gene clusters like Hox genes in animals. Instead, the H3K27me3 mark in Arabidopsis is typically restricted to single-gene bodies [7] , [8] , [9] . Thus, it was well possible that PcG protein-mediated silencing in plants involves different molecular mechanisms and did not involve chromatin compaction. Our DNA inaccessibility data showed global positive correlation between H3K27me3 levels and gene inaccessibility; however, thus, supporting a conserved mechanism of chromatin packaging by PcG proteins in plants and animals. An important question for future studies is whether and how the compact chromatin of the PcG targeted genes is controlled by the plant PcG protein complexes. In addition to genes in constitutive heterochromatin and to PcG protein target genes, we identified a class of inaccessible genes that were very long and had high intragenic CpG methylation. Intragenic CpG methylation was previously found in both mammals [49] and plants [31] , [32] , [33] . It has been proposed that genic DNA methylation results from occasional divergent transcription from cryptic promoters within the gene body that would recruit small interfering RNA-directed DNA methylation activity [31] , [33] . This pathway is possibly distinct from formation of constitutive heterochromatin because CpG methylation in gene bodies is independent of H3K9me2 (refs. 31 , 32 , 33 ). Gene body CpG methylation could interfere with aberrant transcription by restricting access of RNA Polymerase II to intragenic cryptic promoters [31] or by interfering with elongation of RNA P II (ref. 33 ). It is possible that gene body CpG methylation interferes with transcription via chromatin compaction, possibly by recruiting histone deacetylases [4] or by excluding nucleosome-destabilising histone variants [50] . We found in Arabidopsis that long inaccessible genes had lower antisense transcript levels and that DNA methylation was required for low accessibility. These results support a model in which intragenic CpG methylation leads to reduced DNA accessibility, which in turn represses alternative (or cryptic) promoters. Consistent with this notion, sequences at proximal promoters and in the most 5′-region of gene bodies were often excluded from the domain of low accessibility ( Fig. 6a ), suggesting that accessible promoters are needed to sustain transcription of regular transcripts. Facilitating or restricting access to DNA is an ultimate functional output of chromatin, and genome-scale information on DNA inaccessibility is needed for the interpretation of epigenome profiling studies. Our data suggest a complex model of regulation of DNA accessibility. Inactive genes have an intermediate accessibility, which can be greatly reduced by repressive PcG proteins or heterochromatin components. Conversely, transcription is often associated with a local increase in accessibility. For some active genes, increased accessibility is restricted to promoters and 5′-sequences while the accessibility of the largest part of the gene body is strongly reduced by DNA methylation thus preventing transcription from alternative promoters. As DNA methylation was required for reduced accessibility of H3K9me2-marked heterochromatic sequences, we propose that differences in genomic cytosine methylation cause different heterochromatin accessibility between Arabidopsis and Drosophila . Plant material All experiments used Arabidopsis thaliana accession Columbia-0 plants. Plants were grown on soil at 21 °C in darkness (16 h) and at 20 °C in light (8 h). Leaves (leaf no. 6 from ~5 plants per sample) were harvested after 35 days at zeitgeber time 7 (that is, 7 h after start of the photoperiod) and frozen in liquid nitrogen. Note that cell division and expansion had ceased in the harvested leaves. For experiments with reduced DNA methylation, seeds were sown on Murashige and Skoog (MS) plates containing 7 μg ml −1 of 5-azacytidine and grown under long day conditions for 14 days [51] . DNase I-PCR Nuclei from 200 mg of plant material were prepared and treated as described in the Methods section. Five aliquots of 1/8 of the extracted nuclei were subjected to DNase I digestion at final concentrations of 0, 1, 2, 4 and 8 U ml −1 . DNA was extracted from three aliquots of the nuclei using careful phenol–chloroform extraction and ethanol/salt precipitation. Extracted DNA was redissolved in digestion buffer and digested at final DNase I concentrations of 0, 0.25 and 0.75 U ml −1 . DNA recovered from either the digested nuclei or digested DNA was used as template for PCR using specific primers amplifying fragments of about 1.5 kb ( Supplementary Table S1 ). PCR products were quantified using a DNA 7500 kit on the Lab-on-chip platform (Agilent, California), and relative amounts of each fragment were calculated by normalizing to the amount of PCR product from the 0 U ml −1 DNase I-treated samples. To compare the DNA accessibility in plant treated or not treated with 5-azacytidine, nuclei from 25 mg of 14-day old seedlings were subjected to DNase I digestion at final concentrations of 0.05 or 2 U ml −1 . PCR was performed as above. To calculate DNA inaccessibility at the tested loci, PCR product abundance from the 2 U ml −1 DNase I-treated samples was normalized to that from 0.05 U ml −1 -treated samples. The results were then expressed relative to GAPDHα and ACTIN-7 . The experiment was performed in three biological replicates. DNase I-chip We established DNase I hypo-sensitivity profiling based on a published method [52] . Crude nuclei extracts were produced by treating 100 mg of ground frozen plant material in modified nuclei extraction buffer (20 mM PIPES-KOH pH 7.6, 1 M hexylene glycol, 10 mM MgCl 2 , 1 mM ethylene glycol tetraacetic acid (EGTA), 15 mM NaCl, 0.5 mM spermidine, 0.15 mM spermine, 0.5% Triton-X100, 5 mM β-mercaptoethanol and EDTA-free protease inhibitor cocktail (Roche, Switzerland)) for 15 min at 4 °C. The homogenate was filtered through Miracloth (Calbiochem, Germany), and a pellet was collected by a 5-min centrifugation at 1,500 g at 4 °C. Isolated nuclei were washed once in nuclei washing buffer (nuclei washing buffer; 40 mM Tris-HCl pH 8, 0.3 M sucrose, 10 mM MgSO 4 and EDTA-free protease inhibitor cocktail (Roche)) and were used for DNase I (Promega, Wisconsin) digestion for 15 min (final concentration 4.5 U ml −1 for treatment and 0 U ml −1 for background control samples) at 30 °C in digestion buffer (nuclei washing buffer plus 1 mM CaCl 2 ). The reaction was stopped with 50 mM EDTA. The digested nuclei mixture was treated with Proteinase K (Sigma-Aldrich, Missouri) and DNA was extracted using careful phenol–chloroform extraction and ethanol/salt precipitation. Recovered DNA was redissolved and resolved on agarose gels. Gel slabs containing DNA fragments of sizes above 17 kb were excised, and DNA was extracted. The extracted DNA was amplified and labelled using the BioPrime DNA Labelling System (Invitrogen, California). Labelled DNA was hybridized to Affymetrix AGRONOMICS1 Arabidopsis tiling arrays (Affymetrix, Santa Clara, CA) as described [53] . The experiment was performed in three biological replicates. DNase I-chip data analysis All analysis was performed in R [54] . DNase I-chip data were normalized with Model-based Analysis of Tiling-arrays (MAT) [55] implemented in the Aroma Affymetrix package [56] with the window size parameter set to 500. Inaccessible regions were defined as continuous runs of probes with a MAT score of at least three and were selected using the package Bayesian Analysis of ChIP-chip experiments (BAC) [57] with minRun and maxGap parameters set to 5,000 and 200, respectively. Hyper-accessible regions were identified similarly as continuous runs of probes with a MAT score of not > −8 and with minRun and maxGap parameters set to 100 and 200, respectively. Genomic features such as genes and TEs were considered to be part of an enriched region when the region covered at least half of the feature’s length. A gene-specific MAT score was defined as the trimmed mean (trimming the 5% most extreme values) of all probe-specific MAT scores for the probes located entirely within the transcribed region of a gene. Only genes interrogated by at least three-specific probes were considered. Bioinformatic analysis Visualization of tiling array data was done using the Integrated Genome Browser [58] . H3K27me3, H3K9me2 and DNA methylation data were from published results [8] , [53] , [59] . All P -values for differences between median values of gene sets were calculated using Wilcoxon’s-signed rank test. Transcript profiling RNA was extracted, labelled and hybridized to Affymetrix Arabidopsis AGRONOMICS1 microarrays as described [60] using the GeneChip Whole Transcript Sense Target Labelling Assay (Affymetrix). Summarized gene transcript abundances were derived using the Robust Multi-array Average (RMA) algorithm as described [53] . Summarized gene antisense transcript abundances were derived similarly, using the probes from the antisense strand [60] . Strand-specific RNA-seq data were obtained from Gene Expression Omnibus (GEO) (accession code GSM277612 (ref. 41 )). Counts of reads with perfect matches to the antisense strand between transcriptional start and end of annotated genes were normalized to gene lengths. For gene expression profiling by reverse transcription-quantitative PCR, total RNA was extracted from 14-day old seedlings using ISOL-RNA Lysis reagent (5 Prime, Germany) and depleted for genomic DNA using RQ1 RNase free DNase I (Fermentas). First strand cDNA was synthesized using RevertAid First Strand cDNA Synthesis Kit (Fermentas, Germany). Transcript abundance was detected using quantitative PCR with TaqMan Gene Expression Master Mix (Life Technologies, California) and probes from the Universal Probe Library (Roche, Switzerland). Oligonucleotide sequences are listed in Supplementary Table S1 . Transcript abundance of genes was normalized to that of GAPDHa and ACTIN-7 . The experiment was performed in three biological replicates. Accession codes : Microarray data have been deposited in ArrayExpress under accession code E-TABM-1219 . How to cite this article: Shu H. et al . Distinct modes of DNA accessibility in plant chromatin. Nat. Commun. 3:1281 doi: 10.1038/ncomms2259 (2012).